Structure–dynamics relationship in coherent transport through disordered systems Quantum transport is strongly influenced by interference with phase relations that depend on the scattering medium. As even small changes in the geometry of the medium can turn constructive interference to destructive, a clear relation between structure and fast, efficient transport is difficult to identify. Here we present a complex network analysis of quantum transport through disordered systems to elucidate the relationship between transport efficiency and structural organization. Evidence is provided for the emergence of structural classes with different geometries but similar high efficiency. Specifically, a structural motif characterized by pair sites, which are not actively participating to the dynamics, renders transport properties robust against perturbations. Our results pave the way for a systematic rationalization of the design principles behind highly efficient transport, which is of paramount importance for technological applications as well as to address transport robustness in natural-light-harvesting complexes. Transport of charge or energy through disordered landscapes is one of the most fundamental mechanisms underlying biological and technological functionality [1] , [2] , [3] . If the entities that are being transported behave wave-like, that is, propagate coherently, interference resulting from scattering off the disordered medium can result in strong focusing behaviour due to constructive interference, as observed, for example, for an electron gas [4] , the coherent back-scattering of light from atomic clouds [5] and predicted for Bose–Einstein condensates [6] . When this focus lies in the region to which an object should be transmitted, coherent behaviour results in enhanced transport as compared with incoherent (particle-like) processes [7] , [8] . Consequently, it would be highly desirable to exploit such enhanced transport mechanisms. Constructive interference, however, relies on well-defined phase relations that need to be satisfied rather accurately, but get easily altered due to small changes in the geometry of the scattering medium. The onset of destructive interference then reduces transport, or suppresses it completely [9] . This results in a highly complicated structure–functionality relationship: two structures with hardly noticeable geometric differences can lead to strongly different transport properties, and two structures with similar transport properties might not share any geometric similarity. It is thus rather hard to identify geometric features associated with good transport, what would be absolutely necessary for the use of constructive interference as design principle in technological applications. The inherent complexity of the problem as well as the large number of degrees of freedom involved calls for the application of advanced statistical tools. Inspired by the substantial achievements of network science to elucidate complex systems like, for instance, economic growth [10] , human diseases [11] and organic chemistry [12] , our aim is to shed light on the elusive relationship between the structure of disordered media and constructive interference. This is achieved by complex network analysis of quantum transport through disordered system, which allows us to identify a clear structural motif formed by pair sites that are not actively involved in the dynamics, but provide both enhancement of transport and robustness against random displacement of the sites. Our results can be used as a starting point to address robustness of transport in natural systems like light-harvesting complexes. The quantum transport model We consider a discrete two-level N -body system, whose interactions are described by a tight-binding Hamiltonian where describe the annihilation/creation of an excitation at site i , J is the coupling constant and r 0 defines the natural length scale of the system. The interaction rate decays cubically with the distance between the sites in accordance with dipole–dipole interaction. Within this model a structure is defined by the positions of the N sites. The initially excited site (input) and the output site where the excitation has to be delivered are located at diagonally opposite corners of a cube of side r 0 , whereas the remaining N −2 sites are placed at random positions within this cube. Although we looked at systems with N ranging from 4 to 8, most of our attention focused on N =6, being the smallest set for which non-trivial behaviour emerged. For this case, a large sample of 100 million random structures was generated. This sample covered the whole spectrum of transport efficiencies ε , where ε is defined as the maximal probability to find the excitation at the output site within a short time interval after initialization. To make sure that we exclusively target fast transport that necessarily needs to result from constructive interference, we chose , that is, a time-scale that is ten times shorter than the scale associated with direct interaction between input and output sites [13] (see Supplementary Note 1 for further details). Being interested in the characterization of efficient transport, our analysis focused on structures with ε >0.9, a property that is satisfied by only 14,280 configurations out of the generated 10 8 . From a structural point of view this reduced set is highly heterogeneous, meaning that two structures with similar efficiency do not necessarily share any evident common pattern [13] . Such structural variety hinders a straightforward interpretation of the geometrical features compatible with efficient transport. The quantum efficiency network To unravel this structure–dynamics relationship, we applied a set of tools based on complex networks originally developed for the characterization of molecular systems [14] , [15] . Specifically, these methods are designed to analyse large ensembles of configurations, potentially allowing in this case a systematic classification of structures that lead to exceptional transport. We generated a complex network where the 14,280 structures with ε >0.9 represent the nodes, and a link is placed between them if two structures are geometrically similar independently on the specific dynamics of the excitation. The parameter used to estimate structural similarity is , where is the distance between corresponding sites in any two structures. Links were placed when (see Methods for further details on the network creation protocol). The resulting quantum efficiency network is shown in Fig. 1a . In this picture, nodes are proportionally close in space according to the amount of common neighbours. The colour coding adopted for this network will be discussed in detail below, anticipating at this stage that the presence of densely connected regions, that is, clusters of nodes that are highly interconnected among each other, indicates the presence of groups of structures with common geometrical motifs. 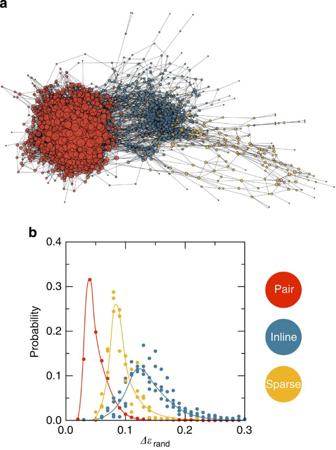Figure 1: The quantum efficiency network. (a) Nodes in the network represent structures with six excitable sites (N=6) andε>0.09. Links are placed if two structures are geometrically similar. The network layout is obtained via the Fruchterman–Reingold algorithm25, which puts nodes with several neighbours in common close in space. To avoid overcrowding in the network layout, only one-fifth of the nodes have been represented in the picture. Node size is proportional to the number of links. (b) The probability distribution of efficiency loss upon random displacements for the eight clusters (calculated on the whole sample, see main text for details). All eight distributions are shown where colours are chosen to highlight the presence of three classes (lines are a guide to the eye). Network nodes colour coding follows the class definitions: pair (red), inline (blue) and sparse (yellow). Figure 1: The quantum efficiency network. ( a ) Nodes in the network represent structures with six excitable sites ( N =6) and ε >0.09. Links are placed if two structures are geometrically similar. The network layout is obtained via the Fruchterman–Reingold algorithm [25] , which puts nodes with several neighbours in common close in space. To avoid overcrowding in the network layout, only one-fifth of the nodes have been represented in the picture. Node size is proportional to the number of links. ( b ) The probability distribution of efficiency loss upon random displacements for the eight clusters (calculated on the whole sample, see main text for details). All eight distributions are shown where colours are chosen to highlight the presence of three classes (lines are a guide to the eye). Network nodes colour coding follows the class definitions: pair (red), inline (blue) and sparse (yellow). Full size image We identified these regions using a network clusterization algorithm based on a self-consistency criterion in terms of network random walks [15] , [16] (see Methods ) that split the network into eight clusters comprised of structures with similar site arrangements. The eight clusters have very different relative populations, 73.3%, 9.2%, 4.7%, 3.2%, 2.6%, 1.9%, 1.2%, 1.1%, respectively. As such, there is a bias towards certain structure types with respect to others. Cumulatively the eight clusters represent the 97% of the whole sample with an unclassified 3% due to noise (see Supplementary Fig. S1 ). Efficiency loss upon random displacement The detection of eight clusters does not imply the presence of eight distinct dynamical behaviours. We therefore probed transport robustness against random displacements of the individual sites of a structure, with displacements restricted to a cube of side 0.05 r 0 centred around the original position of the site. For each structure, was calculated as the original efficiency minus the average efficiency obtained from 1,000 site randomizations. In this scheme, structures were kept rigid under the assumption that the dynamics occur on a much faster time scale than low-frequency fluctuations of the entire system (for example, in the context of biological systems this would be equivalent to large-scale protein breathing). The distributions of for the eight clusters are shown in Fig. 1b . Strikingly, the data spontaneously grouped into three distributions that are coloured in red, blue and yellow in the figure. This coding split the network in homogeneously coloured parts, as shown in Fig. 1a . This was a priori not obvious as the network could have shown a certain degree of colour mixing, providing strong evidence that network topology and excitation dynamics are correlated properties. Summarizing, the random displacements analysis provided evidence that all structures within a cluster show similar response upon perturbation and that three well-defined types of responses emerge from the eight clusters. Classes of quantum behaviour These results suggested a characterization of the whole sample of efficient structures into three classes of similar quantum behaviour. The classes are named ′pair′, ′inline′ and ′sparse′ because of their average geometrical properties. In fact, they show couples of sites very close to each other, a compact arrangement around the input/output axis and a more sparse geometry, respectively. In terms of clusters, the pair class includes only one cluster (the most populated one, 73.3% of the whole sample), whereas the inline includes four clusters (17.6%) and the sparse only three (6.3%). The pair class is very robust against random displacements, with an average loss of efficiency of around 0.06 (red data in Fig. 1b ). Interestingly, this class performed much better than the inline and sparse classes, which showed an average loss of 0.14 and 0.10, respectively (with losses up to 0.3 for the former). These results indicated that the geometry in these latter classes is more correlated, whereas in the pair class sites can be moved by small displacements in an independent fashion. However, robustness comes with a price: the pair class is generally slower. For the fastest processes in each class, the times at which the population in the output site is maximal are 0.67, 0.30 and 0.54 τ for the pair, inline and sparse class, respectively, whereas in average these values are of 0.92, 0.83 and 0.86 τ for the three classes, respectively. In Fig. 2 several properties of the three classes are illustrated. On the left side of the picture structures belonging to the cluster with highest efficiency within the class are overimposed on top of each other (see Supplementary Figs S2 and S3 for the remaining ones). This representation allows a visual appreciation of the structural homogeneity within a cluster as well as of the diversity among clusters. In the right part of the picture, the exciton dynamics of the most efficient structure of the class is shown. In all three cases transport efficiency is larger than 0.97. However, the three dynamics differ substantially. In the pair class (right part of Fig. 2a ), two of the intermediate sites are successively excited with no active role for the other sites (excluding input and output). Conversely, the other two classes show more complex patterns of excitation. These results provide evidence for a strong structure–dynamics relationship given that the final values of the efficiency are very similar in all three cases. 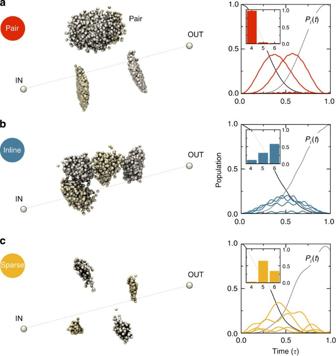Figure 2: Structure–dynamics relationship for selected classes. (a) Represents pair, (b) an inline and (c) sparse classes. On the left side of the figure, structures belonging to the cluster containing the most efficient configuration of the class are overimposed (namely cluster number 1, 2 and 7, respectively, seeSupplementary Figs S2 and S3for the remaining ones). Characteristic structural motifs emerge from each of the different clusters. The exciton dynamics of the most efficient structure of each class is shown in the right part of the figure where thexandyaxis represent the time and the excitation probability (population), respectively. Input and output sites are shown as black and dark grey lines. The relative frequencies to find structures with four, five or six active sites (including input and output sites) within each class are shown as insets (see main text for details). Sites are coloured alternatively in light and dark grey to highlight their different positions. Structural rendering was done with VMD24. Figure 2: Structure–dynamics relationship for selected classes. ( a ) Represents pair, ( b ) an inline and ( c ) sparse classes. On the left side of the figure, structures belonging to the cluster containing the most efficient configuration of the class are overimposed (namely cluster number 1, 2 and 7, respectively, see Supplementary Figs S2 and S3 for the remaining ones). Characteristic structural motifs emerge from each of the different clusters. The exciton dynamics of the most efficient structure of each class is shown in the right part of the figure where the x and y axis represent the time and the excitation probability (population), respectively. Input and output sites are shown as black and dark grey lines. The relative frequencies to find structures with four, five or six active sites (including input and output sites) within each class are shown as insets (see main text for details). Sites are coloured alternatively in light and dark grey to highlight their different positions. Structural rendering was done with VMD [24] . Full size image Inactive pair sites enhance transport The pair class shows a prototypical modular structure. The first module is comprised of four sites including the input and output approximately lined up along the input/output axis, defining a backbone for the entire structure (light grey spheres in Fig. 3a ). The second module is formed by the remaining two sites, the pair (dark grey spheres). Backbone sites are approximately equally spaced between input and output with typical inter-sites distances of ~0.60−0.64 r 0 . Pair sites instead are always very close to each other with a inter-site distance of around 0.25 r 0 (see Supplementary Fig. S4 ). 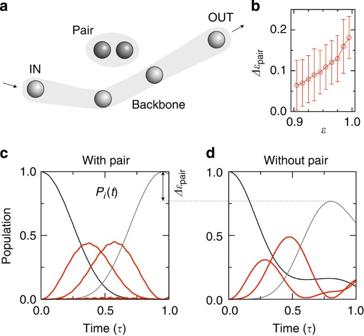Figure 3: Characterization of the pair class. (a) The most efficient structure: pair and backbone sites are shown in dark and light grey, respectively. (b) Efficiency loss upon pair removal as a function of the original efficiencyε. Error bars are calculated according to the standard deviation. (c,d) Comparison of the typical dynamics with and without the pairs. The coherent signal does not focus in the output site in the absence of the pair sites, resulting in an efficiency lossof up to 0.32 (in the plot the dynamics of the most efficient structure is shown, where). Figure 3: Characterization of the pair class. ( a ) The most efficient structure: pair and backbone sites are shown in dark and light grey, respectively. ( b ) Efficiency loss upon pair removal as a function of the original efficiency ε . Error bars are calculated according to the standard deviation. ( c , d ) Comparison of the typical dynamics with and without the pairs. The coherent signal does not focus in the output site in the absence of the pair sites, resulting in an efficiency loss of up to 0.32 (in the plot the dynamics of the most efficient structure is shown, where ). Full size image The position of the pair is more heterogeneous than the backbone sites, that is, their position in space changes between structures as indicated by the disperse cloud of sites in the structural overlaps of Fig. 2a . A first indicator of the origin of the increased robustness is then given: pair sites can be moved within a larger volume without dramatically affecting the transport efficiency ( Supplementary Fig. S4 ). Backbone and pair sites show a completely different dynamical behaviour. Systematic analysis of the distribution of the maximum excitations per site within the pair class (excluding input and output sites) revealed that backbone and pair sites can be clearly divided into ‘active’ and ‘inactive’ exciton carriers, respectively (see Supplementary Fig. S5 ). In fact, backbone sites present maximum excitation probabilities always larger than 0.25, whereas pair sites never more than 0.075 in 99% of the cases. Strikingly, removal of the pair from the original structures resulted in a systematic efficiency loss of up to 0.32, which is rather surprising given that pairs hardly serve as carriers of the excitation. Efficiency loss is particularly severe for the most efficient realizations due to the sensitivity of perfect constructive interference against perturbations ( Fig. 3b ). Pair removal affects exciton transport in non-trivial ways as shown by the quantum dynamics of the most efficient structure before and after pair removal (see Fig. 3c,d ). In the modified structure, we found unbalanced transport along backbone sites contrary to what was originally observed as well as an inability of the input site to promptly transmit the excitation to the closest backbone site. To investigate the mechanism behind the dynamical influence of the pair, we compared the distribution of the energy eigenvalues with and without the two pair sites. Given the weak interaction between the backbone and the pair, there are N −2 eigenstates with the excitation localized on the backbone; in the remaining two eigenstates the excitation is delocalized on the pair symmetrically (antisymmetrically), that is, in the form of a triplet (singlet) state . As depicted in Fig. 4 , the interaction between the backbone and the pair sites results in a shift of the eigenfrequencies of the former N −2 eigenstates (denoted by λ i ( ) in Fig. 4 and Supplementary Figs S6 and S7 , such that their differences are close to integer multiples of a fundamental frequency. With this shift, the excitation is transferred to the output site essentially perfectly after one period of this fundamental frequency. The frequency shift results from a coupling between the former N −2 eigenstates and the triplet state; perturbatively it reads , where v is the interaction between backbone and the pair and δ is the interaction between the two pair sites, that is, the eigenfrequency of the triplet. As all coupling elements in (1) have the same distance-dependence ( ), the energy shift is roughly independent under a change of the backbone-pair distance by a factor of α and a simultaneous change of the pair-size by a factor α 2 . This expectation is explicitly verified in the Supplementary Fig. S4d , where a broad parabolic plateau of high efficiency is clearly discernible (yellow area). Only for small backbone-pair distances in the non-perturbative regime the plateau breaks down ( Supplementary Fig. S7 ). The robustness with respect to perturbations and the resulting statistical significance of the pair mechanism can also readily be deduced from the perturbative mechanism. As a loss of efficiency due to a change of distance between the backbone and the pair can be compensated by a change in the distance between the pair sites, there is not a unique or discrete set of optimal spatial configurations, which one would have otherwise expected for a mechanism based on constructive interference of many paths. Instead, what is found is a higher-dimensional manyfold of optimal configurations. 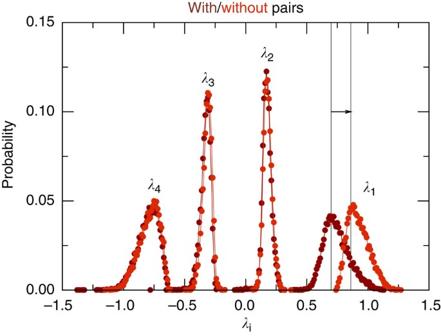Figure 4: Shift of eigenfrequencies due to interactions between backbone and pair sites. Distribution of eigenvaluesλin the presence or absence of interaction with the pair in the first cluster (in red and dark red respectively). In the presence of the pair the differences of theλiare close to integer multiples of a fundamental frequency (seeSupplementary Fig. S6). Figure 4: Shift of eigenfrequencies due to interactions between backbone and pair sites. Distribution of eigenvalues λ in the presence or absence of interaction with the pair in the first cluster (in red and dark red respectively). In the presence of the pair the differences of the λ i are close to integer multiples of a fundamental frequency (see Supplementary Fig. S6 ). Full size image From a geometrical point of view the pair class provides attributes commonly observed in models with different number of sites. For N =4 the ensemble of structures with ε >0.9 organized on a line with inter-site spacings very similar to the ones found in the backbone of the pair class. This is shown in Fig. 5 by superimposing the most efficient structures for N =4 and N =6 (light blue and grey spheres, respectively). However, the maximum efficiency for N =4 is of only 0.922, whereas the presence of pair sites lead to a maximum efficiency of 0.998, which is also the best value achieved within the whole sample of 100 million structures. The general role of pairs is confirmed by the N =8 case. In this model roughly half of the whole sample with ε >0.9 presented a modular structure with four out of eight sites organized in two pairs with the remaining sites perfectly overimposed to the backbone of N =6 (green spheres in Fig. 5 ). Such geometry clearly represents a generalization of the pair class. The pair structure was also observed with N =7, where the backbone was formed by five equidistant sites. Altogether, these results provided strong evidence that pair sites have an important structural role to tune up quantum efficiency, suggesting the idea that they represent a general building strategy towards efficient transport in multi-body quantum systems. 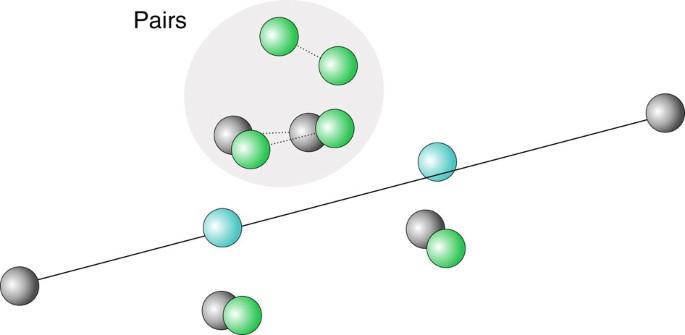Figure 5: Geometries with efficient quantum transport for different numbers of sites. The most efficient structures in the caseN=4 (ε=0.922),N=6 (ε=0.998) andN=8 (ε=0.993). The three cases are shown in light blue, grey and light green, respectively. The grey area highlights the presence of pairs forN=6 andN=8. Figure 5: Geometries with efficient quantum transport for different numbers of sites. The most efficient structures in the case N =4 ( ε =0.922), N =6 ( ε =0.998) and N =8 ( ε =0.993). The three cases are shown in light blue, grey and light green, respectively. The grey area highlights the presence of pairs for N =6 and N =8. Full size image The presence of active and inactive carriers of the transport efficiency in the pair class pointed out a potentially intriguing scheme to rationalize the quantum dynamics of all classes ( Supplementary Fig. S5 ). Taking 0.075 as a threshold to define a site as inactive, the pair class is characterized by a total of four active sites including the input and output (see probability distribution of active sites in the inset of Fig. 2a ). However, for the inline and sparse classes no clear separation into number of active sites was found (inset plots in panel (b) and (c) of Fig. 2 , respectively, see also Supplementary Fig. S5 ). Moreover, when this concept was used for the analysis of the efficiency loss upon random displacements by grouping structures according to the number of active sites, ambiguities raised between the five and six active sites groups due to strong overlaps (see Supplementary Fig. S8 ). These results indicated that the active site concept alone is not sufficient to define structural groups with similar dynamics, reiterating the idea that advanced techniques for structural comparisons, like the one performed here, are necessary to unravel the connection between structure and quantum dynamics. The incoherent case All the presented analysis was performed with perfectly coherent dynamics. The impact of noise on our analysis was investigated by considering environmental models leading to both Markovian and non-Markovian dynamics (see Supplementary Note 2 for details). Within each case, addition of noise consistently decreased the efficiency with no specific distinction among the three classes, most importantly without affecting the response to random displacement classification identified with coherent dynamics (see Supplementary Figs. S9 and S10 ). The purely destructive effect of noise is consistent with the type of analysis performed, which focused on outstandingly fast and efficient transport made possible only by constructive interference [17] . This represents a different scenario with respect to problems where environmental noise can have a beneficial effect [18] , [19] , [20] , [21] . In conclusion, our work provided strong evidence for the emergence of non-trivial characteristic structural motifs leading to high-quantum transport efficiencies. Specifically, the identification of site pairs that do not participate directly to the exciton dynamics results in a general strategy to both enhance quantum efficiency and to make structures robust against geometric perturbations. Consequently, a design principle is presented, exploiting enhanced quantum transport in cases where perfect interferometric stability is impossible. Gaining control on this problem is of paramount importance towards the rational design of technologies making use of constructive interference. The analysis of the pair class led to the identification of a modular arrangement of the dynamics within these structures: an active four-site backbone accompanied with an inactive pair. Such a modular active/inactive arrangement of the excitation dynamics has been also identified in natural-light-harvesting complexes like Fenna-Matthews-Olson (FMO) [22] . The seven chromophores can be divided in two weakly interacting sets, corresponding to an approximately block-like structure of the Hamiltonian [23] : chromophores 1 and 2 are strongly coupled to each other, and weakly with the remaining sites excluding the output number 3. This entails that, upon excitation of chromophore 6 (one of the two supposed entry points of the excitation from the antenna), the chromophores 1 and 2 seem to be effectively decoupled from the dynamics, just as the pairs in our system, but might still analogously influence the dynamics. There are, however, a number of differences that must be kept in mind when comparing the results of the present work with natural-light-harvesting complexes. At a fundamental level, the ratio behind the definition of efficient transport follows from a different perspective, namely transfer being lossless in the FMO and fast in this work. Furthermore, care is needed when comparing geometries of a network of point-like entities with distance based coupling with a much more complicated pigment–protein complex. In light of these differences a straightforward identification of geometric arrangement akin to the pair class in realistic natural systems should not be expected. In other words, in the two systems we find a similar modular arrangement of the dynamics, which, due to the differences in the model, does not necessarily arise from similar geometrical arrangements. Network creation Network links are put according to a similarity parameter. The similarity parameter S is calculated as: where d i is the distance between corresponding sites and i runs over all six sites. The sites are indistinguishable, thus all different permutations of the site labels need to be performed (in number of ( N −2)!, excluding input and output). In addition, symmetry along the in–out axis and an additional mirror symmetry has to be taken into consideration. The measure S between configurations A and B is calculated as follows: keeping fixed the set of labels for A, the labels of B are changed. For each of these ( N −2)! sets, 180 rotations of 2° each of the configuration B are done around its in–out axis. For each rotation, a mirror reflection relative to the x − y =0 plane is also done. The final value of S is then the minimum value of among the ( N −2)! × 180 × 2 possible combinations of labels, rotation and mirror states. Only S 2 values < are considered as links in the network. That means, the average d i between sites of two superimposed configurations must be < . This value lies just above the tail of the pairwise distance distribution (inset Supplementary Fig. S11a ). Consequently, only the most similar structures are linked together. Lower values of the cut-off would generate a disconnected network, whereas values too close to the maximum of the distribution would put links between structures that are not very similar. A double check with another cut-off value of was performed, giving results very similar to the ones shown in the main text (see Supplementary Fig. S11b,c ). Although the change from to seems negligible, it is worth noticing that it corresponds to an increase in the total number of links from 1.03 × 10 6 to 1.42 × 10 6 , that is, a considerable 40%. Clusterization procedure To obtain different homogeneous classes of configurations, the Markov cluster algorithm (MCL) was used [15] , [16] . This algorithm is based on the behaviour of random walks on the network and consists of four steps: (i) start with the transition matrix C of the network, where each column is normalized to one; (ii) compute C 2 ; (iii) take the p th power ( P >1) of every element of C 2 , normalizing afterward each column and (iv) go back to step (ii). After some iterations MCL converges to C MCL , where only few entries for each column are non-zero (exactly only one non-zero entry per column). These entries give the clusters. The parameter p is related to the granularity of the clustering process. High values of p generate several small homogeneous clusters. On the other hand, in the limit of P =1, only one cluster is detected. In this work P =1.4 was used, giving a very good signal-to-noise ratio (see Supplementary Fig. S1 ). Smaller values of P gave similar results. For instance, P =1.2 splits the network into two clusters: the one corresponding to the pair class described in the main text and the remaining two classes all together. This suggests that differences between the clusters in inline and sparse classes appear at a finer degree of granularity, whereas separation between these and the pair class is more evident, requiring a lower parameter P to be resolved. Structural superposition Figure 2 and Supplementary Figs. S2 and S3 are obtained as follows: for each cluster, the most connected structure is taken as reference and all the others are superimposed to that. For each of them the combination of labelling, rotation and mirror state which minimizes the similarity parameter S was taken (see Network creation section). To reduce noise, the coordinates of the sites were averaged with the ones from two other structures of the cluster taken at random. Structural rendering was done with VMD [24] . How to cite this article: Mostarda, S. et al . Structure–dynamics relationship in coherent transport through disordered systems. Nat. Commun. 4:2296 doi: 10.1038/ncomms3296 (2013).